Thermotropic phase boundaries in classic ferroelectrics High-performance piezoelectrics are lead-based solid solutions that exhibit a so-called morphotropic phase boundary, which separates two competing phases as a function of chemical composition; as a consequence, an intermediate low-symmetry phase with a strong piezoelectric effect arises. In search for environmentally sustainable lead-free alternatives that exhibit analogous characteristics, we use a network of competing domains to create similar conditions across thermal inter-ferroelectric transitions in simple, lead-free ferroelectrics such as BaTiO 3 and KNbO 3 . Here we report the experimental observation of thermotropic phase boundaries in these classic ferroelectrics, through direct imaging of low-symmetry intermediate phases that exhibit large enhancements in the existing nonlinear optical and piezoelectric property coefficients. Furthermore, the symmetry lowering in these phases allows for new property coefficients that exceed all the existing coefficients in both parent phases. Discovering the thermotropic nature of thermal phase transitions in simple ferroelectrics thus presents unique opportunities for the design of ‘green’ high-performance materials. High-performance piezoelectric materials are pivotal to modern day ‘smart’ technologies that integrate ultra-sensitive sensing and high-precision actuation functions in biomedical devices, telecommunications and scientific research [1] , [2] . Typically, such smart materials are complex lead-based solid solutions that exhibit a so-called morphotropic phase boundary (MPB), a compositional region separating two competing ferroelectric phases, where an intermediate phase with strongly enhanced functional properties arises [3] , [4] , [5] , [6] . To develop viable alternatives to lead-based piezoelectrics, systems that mimic the principal characteristics [5] , [6] , [7] , [8] of morphotropic phase boundaries (MPBs) have been pursued by means of composition [9] , [10] , pressure [11] , epitaxial strain [12] , [13] , multilayering [14] , [15] and domain microstructure [16] , [17] , [18] . In classic lead-free materials such as BaTiO 3 and KNbO 3 for example, creating frustrated ferroelectric domains by external fields has been shown to substantially enhance piezoelectric response [16] , [17] . However, the exact mechanism of this phenomenon has been the subject of extensive debate in recent years [19] , [20] , [21] , [22] , [23] , [24] , [25] , [26] , [27] ; the possible existence of a monoclinic phase in BaTiO 3 single crystals has been reported [25] , [28] , [29] , but it has never been directly imaged on a microscopic level. As a result, the important question of whether the observed phase is of intrinsic monoclinic symmetry, or in fact corresponds to a symmetry-adaptive superlattice of nano-domains [21] , [30] , [31] , [32] , [33] , [34] , [35] , [36] , [37] (such as those observed in MPBs) remains open. Here we use the mutual interactions inherent to a network of competing domains to create MPB-like conditions across thermal ferroelectric transitions in simple, lead-free ferroelectrics. We provide direct experimental evidence of the resulting intermediate phases of intrinsic monoclinic symmetry using several complementary imaging techniques, while simultaneously mapping their enhanced nonlinear optical and piezoelectric properties on the nanoscale. Thus, we reveal the thermotropic character of thermal ferroelectric phase transitions in classic ferroelectrics. The rationale for this terminology is twofold. On the one hand it draws the analogy to MPBs while emphasizing that here we consider thermal (‘thermo-’) instead of compositional (‘morpho-’) phase boundaries. On the other hand it underlines the similarity to the physics of thermotropic liquid crystals, which exhibit different types of liquid-like orientational order (‘-tropos’) in a certain temperature range [38] . In the following, we focus on the well-known BaTiO 3 and KNbO 3 materials as representative examples of simple, lead-free ferroelectrics. Thermotropic phase boundaries In the bulk, single-domain case, both these perovskite systems undergo a series of first-order ferroelectric transitions upon heating, sequentially adopting rhombohedral (R), orthorhombic (O) and tetragonal (T) ferroelectric phases before reverting to the cubic parent phase (C). In multi-domain configurations, however, phase-field simulations predict the emergence of an intermediate phase if sufficient competing mechanical and dipolar interactions between domains exist. 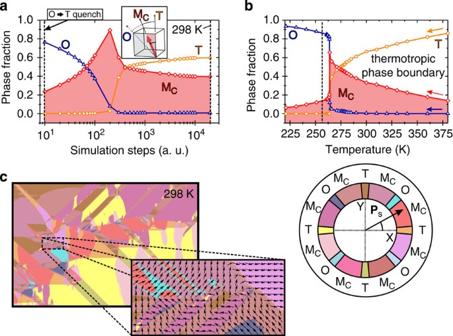Figure 1:Thermodynamically stabilized polarization rotation in multi-domain structures. (a) Volume fractions of orthorhombic (O, open blue triangles), tetragonal (T, open orange circles) and monoclinic (MC, open red diamonds) phases in an orthogonally twinned domain structure, upon quench-heating from 240 to 298 K. The phase classification in terms of discrete ferroelectric polarization (PS) orientation ranges is shown in the legend in (c). (b) Stable volume phase fractions in the orthogonally twinned domain structure as a function of temperature. In both (a) and (b), the red shading acts as a guide to the eye highlighting the evolution of the low-symmetry phase fraction. (c) Selected area of the thermodynamically stabilized domain structure at 298 K. The legend indicates the colour coding of the different ferroelectric phases, as well as their definition in terms of discrete polarization orientation ranges. Inset: zoom-in vector plot of a selected region showing localPSorientations. Figure 1 a shows the temporal evolution of the phase fractions in an orthogonally domain-twinned BaTiO 3 system as it is heated through its O–T phase boundary, calculated using phase-field simulations (see Methods). As can be seen, these simulations predict the emergence of a kinetically intermediate phase of monoclinic (M C ) symmetry [39] which is defined by a spontaneous ferroelectric polarization ( P S ) that significantly deviates (>5°) from the corresponding T and O directions. Moreover, as shown in Fig. 1b , this M C phase is thermodynamically stabilized in significant volume fractions (20–60%) over a wide temperature range of over 100 K. This intriguing reduction of the polar anisotropy [40] is illustrated by the domain structure in Fig. 1c , which reveals a persistent network of bulk M C regions at room temperature (298 K). The thermotropic character of the ferroelectric phase boundary originates from the in-plane shear stress ( σ 23 ) and transverse electric field ( E 2 ) components that are inherently generated by the orthogonal in-plane domain twins, as is evident from their strong spatial correlation with the in-plane polarization rotation angle β ( Fig. 2 , see also Supplementary Note 1 ). Figure 1: Thermodynamically stabilized polarization rotation in multi-domain structures. ( a ) Volume fractions of orthorhombic (O, open blue triangles), tetragonal (T, open orange circles) and monoclinic (M C , open red diamonds) phases in an orthogonally twinned domain structure, upon quench-heating from 240 to 298 K. The phase classification in terms of discrete ferroelectric polarization ( P S ) orientation ranges is shown in the legend in ( c ). ( b ) Stable volume phase fractions in the orthogonally twinned domain structure as a function of temperature. In both ( a ) and ( b ), the red shading acts as a guide to the eye highlighting the evolution of the low-symmetry phase fraction. ( c ) Selected area of the thermodynamically stabilized domain structure at 298 K. The legend indicates the colour coding of the different ferroelectric phases, as well as their definition in terms of discrete polarization orientation ranges. Inset: zoom-in vector plot of a selected region showing local P S orientations. 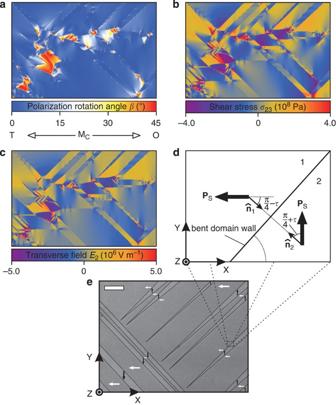Figure 2:Origin of thermotropic phase boundaries. (a) Spatial map of the relative polarization rotation angleβat 298 K, corresponding to the domain structure shown inFig. 1c. Hereβis defined as the absolute deviation from the closest nominal ‹100› polarization axis. (b) Calculated spatial map of the in-plane internal shear stressσ23in the same domain structure. (c) Corresponding map of the calculated in-plane transverse electric field componentE2. As illustrated by the strong spatial correlation betweenβ,σ23, andE2, the polarization rotation finds its origin in the combined effect of the local shear stress and transverse electric field, which is consistent with the experimentally found in-plane shear distortion (see below). (d) Zoomed-in sketch of a slightly bent domain wall, illustrating the mechanism of wall charging upon wall bending (see equation 9 inSupplementary Note 1). The domain wall bending angle is given byτ, and the surface unit normals for domains 1 and 2 are indicated byand, respectively. (e) Optical image (unpolarized incident white light, reflected light polarized along X) of a typical orthogonally twinned multi-domain structure in BaTiO3. Scale bar; 2 μm. Domains are delineated by solid black lines for clarity, arrows indicate proposed polarization directions. Full size image Figure 2: Origin of thermotropic phase boundaries. ( a ) Spatial map of the relative polarization rotation angle β at 298 K, corresponding to the domain structure shown in Fig. 1c . Here β is defined as the absolute deviation from the closest nominal ‹100› polarization axis. ( b ) Calculated spatial map of the in-plane internal shear stress σ 23 in the same domain structure. ( c ) Corresponding map of the calculated in-plane transverse electric field component E 2 . As illustrated by the strong spatial correlation between β , σ 23 , and E 2 , the polarization rotation finds its origin in the combined effect of the local shear stress and transverse electric field, which is consistent with the experimentally found in-plane shear distortion (see below). ( d ) Zoomed-in sketch of a slightly bent domain wall, illustrating the mechanism of wall charging upon wall bending (see equation 9 in Supplementary Note 1 ). The domain wall bending angle is given by τ , and the surface unit normals for domains 1 and 2 are indicated by and , respectively. ( e ) Optical image (unpolarized incident white light, reflected light polarized along X) of a typical orthogonally twinned multi-domain structure in BaTiO 3 . Scale bar; 2 μm. Domains are delineated by solid black lines for clarity, arrows indicate proposed polarization directions. Full size image To experimentally confirm the thermotropic nature of ferroelectric phase boundaries, we investigate the local symmetry, microscopic structure and properties of these intermediate phases through a variety of complementary nanoscale imaging techniques. Symmetry and nonlinear optical properties Considering that both ferroelectricity and piezoelectricity only occur in materials that lack a structural centre of inversion, we employ nonlinear optical second harmonic generation (SHG)—a second-order process that requires the same lack of inversion symmetry [41] , [42] —to image and assess the local symmetry in these systems. 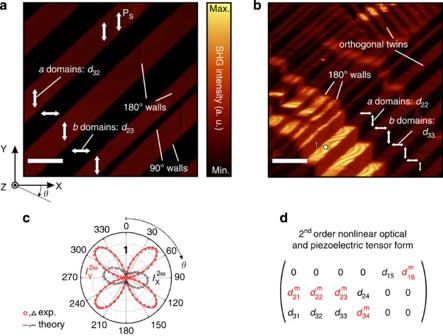Figure 3:Local symmetry imaging and analysis by optical SHG. (a) Scanning SHG microscopy image (with) of an in-planea,b-domain structure in a BaTiO3single crystal without orthogonal twinning. The nonlinear optical tensor coefficients probed in the different domains for this experimental configuration are indicated, and corresponding ferroelectric polarization (PS) axes are marked by double-headed white arrows. The scale bar corresponds to 8 μm. (b) Scanning SHG microscopy image (with) of an in-planea,b-domain structure in a BaTiO3single crystal with orthogonal twinning. Also for this configuration, the polarization axes and active tensor coefficients are indicated. The scale bar corresponds to 12 μm. (c) SHG intensity polar plots ofandcomponents (radius) versus fundamental polarization angle (azimuth angleθ) corresponding to the MCphase. Data points correspond to experiment, and the solid lines correspond to theory based on a monoclinicmpoint group symmetry. (d) Voigt notation form of both the second order nonlinear optical tensor and the piezoelectric tensor, which have the same symmetry attributes42. For tetragonal domains (4mmsymmetry), only the tensor coefficients without superscript (in black) are nonzero, withd24=d15andd31=d32. For monoclinicmsymmetry (min-plane), the tensor coefficients with superscriptm(in red) also become nonzero. Figure 3 compares scanning SHG microscopy images of a BaTiO 3 single crystal in selected areas with and without orthogonal domain twinning. The domain structure in Fig. 3a , comprising only a single set of parallel 90° twin walls, exhibits the typical bright-dark SHG contrast corresponding to in-plane tetragonal a and b domains. As confirmed using spatially resolved SHG polarimetry, their SHG signature seems to adhere perfectly to the nominal tetragonal symmetry of point group 4mm ( Supplementary Fig. 1 ). In contrast, the competition between the two sets of orthogonal twin domains in Fig. 3b induces the anticipated intermediate M C phase, which is characterized by a ‘staircase’ pattern and meandering ripples of strongly enhanced SHG intensity. Local symmetry analysis through SHG polarimetry, Fig. 3c , shows that the point group symmetry in this phase is indeed monoclinic (point group m ), as expected for an M C phase. Independently, this is also confirmed using complementary spatially resolved micro-Raman microscopy (see Supplementary Fig. 2 ). Since the only symmetry element in this point group — the m mirror plane — is parallel to the surface of the crystal, the ferroelectric polarization in the M C phase is symmetry-allowed to continuously rotate in-plane [3] , [4] , [7] , [11] , [43] . In this sense, the bridging M C phase can be regarded as an analogue of a ‘viscous’ two-dimensional polar liquid, with the rotational degree of freedom illustrated by meandering polarization directions. Figure 3: Local symmetry imaging and analysis by optical SHG. ( a ) Scanning SHG microscopy image ( with ) of an in-plane a , b -domain structure in a BaTiO 3 single crystal without orthogonal twinning. The nonlinear optical tensor coefficients probed in the different domains for this experimental configuration are indicated, and corresponding ferroelectric polarization ( P S ) axes are marked by double-headed white arrows. The scale bar corresponds to 8 μm. ( b ) Scanning SHG microscopy image ( with ) of an in-plane a , b -domain structure in a BaTiO 3 single crystal with orthogonal twinning. Also for this configuration, the polarization axes and active tensor coefficients are indicated. The scale bar corresponds to 12 μm. ( c ) SHG intensity polar plots of and components (radius) versus fundamental polarization angle (azimuth angle θ ) corresponding to the M C phase. Data points correspond to experiment, and the solid lines correspond to theory based on a monoclinic m point group symmetry. ( d ) Voigt notation form of both the second order nonlinear optical tensor and the piezoelectric tensor, which have the same symmetry attributes [42] . For tetragonal domains ( 4mm symmetry), only the tensor coefficients without superscript (in black) are nonzero, with d 24 = d 15 and d 31 = d 32 . For monoclinic m symmetry ( m in-plane), the tensor coefficients with superscript m (in red) also become nonzero. Full size image This same degree of freedom is responsible for the observed enhancement of the nonlinear optical coefficients. Depending on the experimental configuration, the SHG scans nominally probe the d 32 and d 33 components of the nonlinear optical tensor of tetragonal BaTiO 3 (see Fig. 3d ). By comparison, in the M C phase, the SHG intensity is found to reach relative values of up to 1,760%, and effective coefficient enhancements of up to 4.2 × and 4.4 × are seen for d 32 (to ≈89 pm V −1 ) and d 33 (to ≈32 pm V −1 ), respectively (see Methods). Moreover, as illustrated in Fig. 3d , the symmetry lowering to point group m results in additional large non-zero nonlinear optical coefficients, which are neither expected nor observed in tetragonal domains: d 22 ≈18 pm V −1 and d 23 ≈22 pm V −1 . We have reproducibly observed the M C phase at room temperature in various BaTiO 3 single crystals from different sources, both before and after annealing at 1,150 K and before and after thermal cycling through the O–T phase boundary. Empirically, it is readily observed whenever orthogonally twinned domain structures are present. Furthermore, an analogous monoclinic phase exhibiting similar SHG enhancements is observed in strongly twinned KNbO 3 single crystals at room temperature ( Supplementary Fig. 3 ), which underscores the generality of the concept of thermotropic phase boundaries in ferroelectrics. In contrast to tetragonal BaTiO 3 , KNbO 3 is nominally orthorhombic at ambient temperatures, where it is situated closest to the R–O phase boundary. Structure There are prior reports of an intermediate M C phase near the thermal O–T phase boundary of BaTiO 3 . Cao et al. [28] reported on a M C phase at 265 K, discovered after cooling BaTiO 3 single crystals through the T–O transition under an applied electric field. Recently, Eisenschmidt et al. [29] observed monoclinic M C -type short range order while slowly cooling BaTiO 3 single crystals through the same transition. However, both these works employed conventional X-ray diffraction techniques, wherein many ferroelectric domains are probed simultaneously due to the large size of the X-ray beam. As a result, neither work could experimentally determine whether the observed low-symmetry stems from an intrinsically monoclinic structure, or from a domain-averaged adaptive superlattice consisting of nanotwinned parent-phase domains [21] , [30] , [31] , [32] , [33] , [34] , [35] , [36] , [37] (see Supplementary Note 2 ). Here we experimentally demonstrate the natural occurrence of a bulk, long-range ordered M C phase in unpoled BaTiO 3 at room temperature; at considerable distance from the thermal O–T phase boundary. Moreover, by employing a state-of-the-art focused beam diffraction technique, scanning X-ray diffraction microscopy (nano-SXDM [44] , [45] ), we show below that the observed M C phase is an intrinsically monoclinic structure, as opposed to a consequence of hypothetical nanoscale domain twinning. Nanoscale SXDM measurements reveal that the (220) diffraction corresponding to the M C structure appears as a newly observed peak close to the (220) diffraction peak of tetragonal b domains ( Fig. 4a–c ). Owing to the intentional shadowing of the focused beam centre in SXDM, each Bragg diffraction peak typically appears as two vertically separated lobes, whose angular centre of mass reflects the corresponding (2 θ , χ ) coordinate ( Supplementary Fig. 4 ) [44] , [45] . The extended area diffraction image in Fig. 4a demonstrates that the observed M C diffraction cannot be due to conventional diffraction from coarse tetragonal or orthorhombic domain twins, as any such reflection would fall well outside of the experimental zoom-in window used throughout our imaging experiments (see also Supplementary Note 2 ). Moreover, a possible nanotwinning origin can be ruled out as unphysical, as the position of the M C diffraction peak violates both the reciprocal space lever rule [35] , [36] , [37] ( Fig. 4d and Supplementary Figs 5–7 ) as well as the general invariance conditions [31] , [32] , [33] of any potential adaptive phase. In addition, both theory [46] , [47] and experiments [48] , [49] , [50] , [51] , [52] demonstrate that the crucial requirement for adaptive phase formation, an extremely low-domain wall energy [31] , [32] , [53] , does not apply in BaTiO 3 at 298 K (see Supplementary Figs 8,9 ). For an in-depth discussion on the exclusion of nanotwinned adaptive phases, see Supplementary Note 2 . 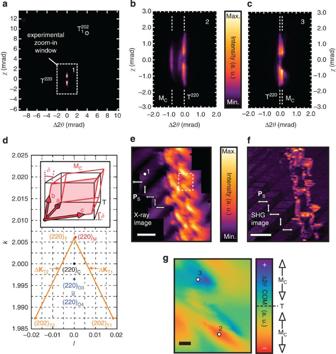Figure 4:Intrinsic shear distortion of the monoclinic MCunit cell probed by nanoscale SXDM. (a) Extended 2D diffraction image of the (220) reflection (T220) from tetragonalbdomains in an orthogonally twinned BaTiO3crystal. The corresponding diffraction positions of coarse tetragonala-domain twins (=(Δ2θ,χ)T1=(3.955, 9.163) mrad and=(Δ2θ,χ)T2=(21.74, 9.163) mrad) or orthorhombic twins (seeSupplementary Note 2) fall far outside the experimental zoom-in window used in our SXDM imaging (dashed white area). (b) and (c) depict background-subtracted, normalized 2D (220) diffraction images corresponding to positions 2 and 3, respectively (seeg). (d) Reciprocal space map comparing diffraction peak positions (kl-plane projections aroundh=2.000) of experimentally observed tetragonal (T) and monoclinic (M) domains to those of hypothetical tetragonal (T1, T2) and orthorhombic (O3,O4) coarse twins. Solid lines ΔKiindicate the lever rules for the diffraction peak positions of potential nanotwinned adaptive phases. Axes are scaled by the reciprocal lattice unit (1.566 Å−1) of cubic (C) BaTiO3at 450 K (ref.28). The inset schematically depicts the MCshear distortion (shearedmmirror plane shaded in red). (e) Aspect-ratio-corrected spatial map of the (220) MCpeak intensity in the orthogonally twinned BaTiO3structure. Scale bar; 10 μm. (f) Corresponding composite scanning SHG image (+awith, whereais scaled to match the SHG intensity in tetragonal domains). Ferroelectric polarization (PS) axes are marked by double-headed white arrows. Scale bar; 10 μm. (g) Zoomed-in high-resolution spatial map (80 nm steps) of Δ2θ=2θ220−2θT,avg.; the difference between the 2θcentre of mass (COM) of the local (220) diffraction signal and the average 2θCOM of an undistorted tetragonalbdomain. Scale bar; 10 μm. Figure 4: Intrinsic shear distortion of the monoclinic M C unit cell probed by nanoscale SXDM. ( a ) Extended 2D diffraction image of the (220) reflection (T 220 ) from tetragonal b domains in an orthogonally twinned BaTiO 3 crystal. The corresponding diffraction positions of coarse tetragonal a -domain twins ( =(Δ2 θ , χ ) T1 =(3.955, 9.163) mrad and =(Δ2 θ , χ ) T2 =(21.74, 9.163) mrad) or orthorhombic twins (see Supplementary Note 2 ) fall far outside the experimental zoom-in window used in our SXDM imaging (dashed white area). ( b ) and ( c ) depict background-subtracted, normalized 2D (220) diffraction images corresponding to positions 2 and 3, respectively (see g ). ( d ) Reciprocal space map comparing diffraction peak positions ( kl -plane projections around h =2.000) of experimentally observed tetragonal (T) and monoclinic (M) domains to those of hypothetical tetragonal (T1, T2) and orthorhombic (O3,O4) coarse twins. Solid lines Δ K i indicate the lever rules for the diffraction peak positions of potential nanotwinned adaptive phases. Axes are scaled by the reciprocal lattice unit (1.566 Å −1 ) of cubic (C) BaTiO 3 at 450 K (ref. 28 ). The inset schematically depicts the M C shear distortion (sheared m mirror plane shaded in red). ( e ) Aspect-ratio-corrected spatial map of the (220) M C peak intensity in the orthogonally twinned BaTiO 3 structure. Scale bar; 10 μm. ( f ) Corresponding composite scanning SHG image ( + a with , where a is scaled to match the SHG intensity in tetragonal domains). Ferroelectric polarization ( P S ) axes are marked by double-headed white arrows. Scale bar; 10 μm. ( g ) Zoomed-in high-resolution spatial map (80 nm steps) of Δ2 θ =2 θ 220 −2 θ T,avg. ; the difference between the 2 θ centre of mass (COM) of the local (220) diffraction signal and the average 2 θ COM of an undistorted tetragonal b domain. Scale bar; 10 μm. Full size image Instead, the (220) M C diffraction is consistent with a simple shear distortion of the tetragonal unit cell that reduces the symmetry to point group m (inset Fig. 4d ). An SXDM rocking curve analysis determines the typical shear angle | δ M | to be ~0.018°, clearly identifying the M C structure as an intermediate phase that bridges the purely tetragonal (| δ T |=0°) and orthorhombic (| δ O |=0.075°) structures [29] (see Supplementary Note 3 and Supplementary Figs 10,11 ). Comparing a spatial map of the integrated intensity of the M C peak ( Fig. 4e ) to the complementary scanning SHG image in the same area ( Fig. 4f ) clearly shows their close correspondence, consolidating the monoclinic origin of the M C diffraction. Furthermore, the micron-scale spatial variation of its 2 θ position (shown in Fig. 4g and Supplementary Fig. 11c ) indicates micron-scale continuous changes of the magnitude and sign of the shear angle δ M within the M C staircase pattern, most likely related to the meandering bright-dark SHG ripples observed in Fig. 2 . We note that δ M does not directly correspond to the rotation of the ferroelectric polarization, which can lie anywhere within the sheared mirror plane. Piezoelectric properties Since the piezoelectric properties near the thermotropic phase boundaries are of specific interest, we measure the local piezoresponse of the M C phase in orthogonally twinned BaTiO 3 ( Fig. 5 ) [54] . As anticipated, both the amplitude ( Fig. 5a ) and phase ( Fig. 5b ) of the piezoresponse in the M C phase are clearly distinct from those in tetragonal BaTiO 3 , which is evident from a comparison with the corresponding scanning SHG image ( Fig. 5c ). Owing to the in-plane domain geometry, the measured vertical piezoresponse corresponds to the voltage-induced in-plane displacement of the sample surface (see Supplementary Note 4 ). As illustrated by the inset in Fig. 5a , a large piezoelectric displacement is induced in the a domains of the M C phase, which is entirely absent in the adjacent tetragonal a domains. This is in excellent agreement with combined phase-field and finite element modelling, which show that this effective displacement arises from a combination of newly induced d 16 and d 22 coefficients ( Supplementary Fig. 12 ). As shown in Fig. 5d , all the piezoelectric d ij coefficients are strongly dependent on the ferroelectric polarization angle, β . For example, by combining experimental and simulation data, we estimate a monoclinic polarization angle of β ≈17° in position 1 of the experimentally observed M C phase, with corresponding values of d 16 ≈69 pm V −1 and d 22 ≈500 pm V −1 ( Supplementary Fig. 12d ). For optimum polarization angles in the M C phase ( β ≈25°), the piezoelectric d 22 coefficient is predicted to peak at ≈840 pm V −1 , which exceeds all existing piezoelectric coefficients of both parent phases. 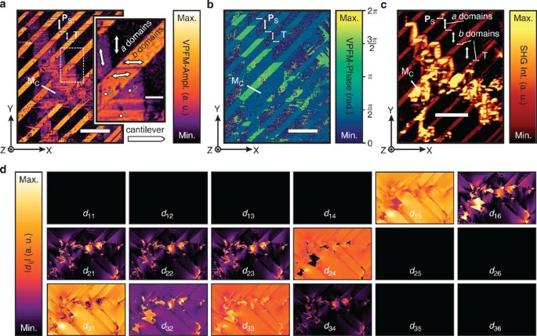Figure 5:Piezoelectric properties in the thermotropic phase boundary of BaTiO3at 298 K. (a) Amplitude image of the vertical piezoresponse as measured by BE-PFM55. The cantilever arm in the measurement was oriented along X. Scale bar; 10 μm. The inset shows a zoom-in on a selected area of the scan (scale bar; 2 μm). (b) Corresponding image of the phase of the vertical piezoresponse. Scale bar; 10 μm. Where the piezoresponse was negligible, the phase was set to 0. (c) Scanning SHG microscopy image (with) recorded in the same area. Here the MCphase is marked by the regions of high SHG intensity. Scale bar; 10 μm. (d) Spatial maps of all phase-field calculated piezoelectric |dij| coefficients corresponding to the orthogonally twinned domain structure inFig. 1c(see Methods). The maps are arranged in Voigt tensor form to allow for direct comparison withFig. 3d. Figure 5: Piezoelectric properties in the thermotropic phase boundary of BaTiO 3 at 298 K. ( a ) Amplitude image of the vertical piezoresponse as measured by BE-PFM [55] . The cantilever arm in the measurement was oriented along X. Scale bar; 10 μm. The inset shows a zoom-in on a selected area of the scan (scale bar; 2 μm). ( b ) Corresponding image of the phase of the vertical piezoresponse. Scale bar; 10 μm. Where the piezoresponse was negligible, the phase was set to 0. ( c ) Scanning SHG microscopy image ( with ) recorded in the same area. Here the M C phase is marked by the regions of high SHG intensity. Scale bar; 10 μm. ( d ) Spatial maps of all phase-field calculated piezoelectric | d ij | coefficients corresponding to the orthogonally twinned domain structure in Fig. 1c (see Methods). The maps are arranged in Voigt tensor form to allow for direct comparison with Fig. 3d . Full size image Our findings reveal that phase transitions in ferroelectrics are intimately coupled to the underlying domain microstructure. Even in lead-free BaTiO 3 and KNbO 3 , classic materials that have been known and studied for over 60 years, we have discovered that domains can lend a thermotropic character to their otherwise well-known phase transitions. This leads to the emergence of intermediate monoclinic phases in a wide temperature range around the conventional ferroelectric transitions. As this phenomenon arises due to the mechanical and dipolar interactions between competing ferroelectric-ferroelastic domains in a complex domain microstructure, advanced nanoscale-resolved multi-technique measurements in the same spatial location, such as those presented here, are required to properly reveal the underlying physics on a microscopic level. We show that in the stabilized intermediate phases, both the piezoelectric and the nonlinear optical properties can be strongly enhanced, and even newly induced. Since the mechanism of symmetry lowering through stresses and fields is in principle universal to non-triclinic ferroelectric crystal systems, these results suggest a host of possibilities for the design of high-performance phases. A fourfold (4 × ) enhancement in functional coefficients from a simple shear strain on the order of 10 −4 indicates that controlled symmetry lowering can indeed be a powerful tool for property enhancement and tuning, and that it does not necessarily require large strains. In this study, a random domain microstructure is shown to inherently generate such strains, thus stabilizing the monoclinic phase. Theory however shows that similar shear stresses and fields, when applied externally to a single domain system, can also generate such monoclinic phases, along with the concomitant property enhancements. Moreover, since symmetry allows the ferroelectric polarization to lie anywhere within the monoclinic mirror plane, m , it is easy to reorient the local polarizations in a polydomain monoclinic system with external fields to achieve a ‘poled’ monoclinic domain microstructure. In addition, the piezoelectric tensor of the monoclinic phase enables shear modes that are particularly suitable for shear mode piezoelectric devices [55] , [56] . Capturing these phenomena using phase-field theory opens the door to predictive modelling of enhanced material properties, and enables the optimization of relevant extrinsic factors such as domain distribution, impurity content and external fields. The fundamental insights presented here will allow for further exploration of strategies to reliably and reproducibly create these high-performance phases through ‘domain-engineering-by-design’. Materials BaTiO 3 and KNbO 3 single crystals (typical size 5 × 5 × 1 mm, {100} pc surface cut) were purchased from Fujian Castech Crystals Inc., China, and Oxide Corporation, Japan. Where necessary, additional polishing of crystal surfaces was performed to obtain satisfactory optical surface quality. Prior to experimental investigation, the samples were cooled through the (T→O) transition to ~240 K in a liquid nitrogen-cooled cryostat and kept there for 1 h. Next, the samples were re-heated to ambient temperature (295 K), resulting in a typical multi-domain structure featuring interpenetrating, orthogonally twinned tetragonal a and b domains. Empirically, we determined that monoclinic signatures were readily found near such orthogonally twinned regions, which typically feature thin, wedge-shaped domains (see Fig. 2e ). These M C signatures were reproducibly observed at room temperature after annealing the sample at 1150 K for 6 h under a 50 cm 3 min −1 O 2 flow, excluding localized sample surface damage as the origin. This is consistent with the observation that Raman imaging using the 514 nm excitation wavelength at higher power densities tends to locally ‘erase’ the monoclinic signatures, which is presumably caused by the locally deposited thermal energy at this wavelength. The energy scale involved in this moderate ‘optical annealing’ process (local heating typically not exceeding the order of 50 K) is sufficient to rearrange the multi-domain structure, while being far below the energy required to induce reconstruction of a potentially damaged crystal surface (local temperatures on the order of 900 K). Furthermore, subsequent thermal cycling of the crystal after such optical erasure readily re-induces the monoclinic signatures. To allow for direct comparison, after thermal cycling the samples were kept at ambient temperature (295 K) in between and during SHG, Raman, nano-SXDM and band-excitation piezoresponse force microscopy (BE-PFM) experiments. Phase-field simulations Our three-dimensional (3D) phase-field model to describe the evolution of the spatial ferroelectric polarization distribution as a function of time is based on the time-dependent Ginzburg–Landau equation where P is the ferroelectric polarization, x is the spatial position in our XYZ Cartesian coordinate system and is the kinetic coefficient related to the domain wall mobility. The total free energy F (a function of the polarization P ) includes all the relevant energetic contributions f : that is, the bulk, gradient, elastic and electrostatic contributions, respectively. The simulations were conducted for BaTiO 3 under stress-free boundary conditions. Stress and strain were calculated from the mechanical equilibrium condition [57] where the σ ij are the stress tensor components. The phenomenological potential and parameters (Landau–Devonshire coefficients, electrostrictive constant and elastic constant tensors) were taken from Li et al. [58] , and the modified isotropic gradient energy coefficients ( g 11 , g 12 and g 44 ) were based on Hlinka et al. [46] The electric field distribution in the multi-domain structure was calculated by first solving the Poisson equation to find the electric potential ϕ (ref. 59 ), and then finding the electric field components through: The discretized quasi-two-dimensional (quasi-2D) simulation size was 1,024Δ x × 1,024Δ x × 4Δ x , with a grid spacing of Δ x =1.8 nm, unless otherwise specified. Periodic boundary conditions were imposed in all three directions. Owing to the quasi-2D nature of the simulations, all domain structures and resulting properties were homogeneous along the out-of-plane -direction. To obtain the orthogonally twinned initial multi-domain structure, we initially seeded two small sets of perpendicular tetragonal twins within the simulation system, filled the rest of the grid with thermal noise and then allowed the system to relax at 380 K until stabilized. The phase diagram in Fig. 1b was constructed by quenching this stabilized 380 K domain structure to a variety of lower temperatures in a set of parallel simulations, evolving the system in each of these until equilibration was reached and plotting the resulting volume phase fractions as a function of the equilibrium temperature. SHG microscopy and polarimetry SHG microscopy and polarimetry were performed in reflection geometry using a modified Witec Alpha 300 S confocal Raman microscope equipped with a 10 nm-resolution XYZ piezo-translation stage. The in-plane ‹100› crystallographic axes of the sample were carefully oriented along the X and Y axes of the experimental coordinate system. A pulsed fundamental beam (Spectra-Physics Tsunami (Ti:Sapphire), λ =800 nm, 80 fs, 80 MHz, chopped at ≈800 Hz) was focused on the sample using a × 100 microscope objective (Nikon, N.A. 0.9) at a typical incident power density of ~100 pJ μm −2 pulse −1 . The lateral spatial resolution was close to diffraction-limited at ≈355 nm (ref. 41 ). The polarization of the fundamental light was controlled by a zero-order half-wave plate mounted in a motorized rotational stage. The second harmonic signal (2 ω ) was collected using the same objective, spectrally filtered and passed through a polarization analyser prior to detection using a Hamamatsu R928 photo-multiplier tube. Nonlinear optical d ijk coefficients were calculated using reference values for tetragonal BaTiO 3 taken from Miller et al. ’s early work [60] , [61] , which were scaled using Miller’s Δ (which is assumed invariant for the SHG process in the same material [62] , [63] ): Here, ω 3 = ω 1 + ω 2 represents the SHG process, and the n i ( ω ) are the appropriate ordinary and extraordinary refractive indices of single domain BaTiO 3 at 295 K, as calculated using the known Sellmeier coefficients [64] . Induced nonlinear optical d ijk coefficients were estimated by linear multiplication of these scaled d ijk coefficients for tetragonal BaTiO 3 and the appropriate SHG intensity ratios (that is, d ijk ratios are taken the same as appropriate SHG intensity ratios obtained from the same scan). Note that both the nonlinear optical and piezoelectric tensors are third-rank polar tensors, and therefore subject to the same symmetry restrictions [42] . However, although they are also similarly labelled as d , they describe very different physical phenomena. All SHG experiments described in this work were performed in air, at ambient pressure and temperature (1 atm, 295 K). Monoclinic signatures were monitored as a function of time after thermal cycling and found to be stable up to at least 6 months when samples were kept at 295±2 K. Raman microscopy Raman microscopy was performed in reflection geometry on the same modified Witec Alpha 300 S confocal Raman microscope. The in-plane ‹100› crystallographic axes of the sample were carefully oriented along the X and Y axes of the experimental coordinate system. The continuous wave 514.5 nm excitation beam (Melles Griot 43 Series Ar + -laser) was focused on the sample using a × 100 microscope objective (Nikon, N.A. 0.9) at a typical incident power density of about 1 mW μm −2 (lateral spatial resolution ≈350 nm (ref. 41 )). The polarization of the excitation light was controlled by a zero-order wave plate mounted in a rotational stage. The scattered Raman signal was collected using the same objective, spectrally filtered using an edge-pass filter (Semrock Inc.), and detected using an Acton Spectra-Pro 2300i monochromator equipped with a thermoelectrically cooled Andor DV401 CCD array. All Raman experiments described in this work were performed in air, at ambient pressure and temperature (1 atm, 295 K). Nanoscale scanning X-ray diffraction microscopy Nanoscale Scanning X-ray Diffraction Microscopy (nano-SXDM) experiments were performed using the Hard X-ray Nanoprobe (HXN) of the Center for Nanoscale Materials (CNM) at sector 26-ID-C of the Advanced Photon Source, Argonne National Laboratory. The coherent and monochromatic incident X-ray beam (photon energy 10.0 keV, λ =1.2398 Å) was focused on the sample by a Fresnel zone plate (Xradia Inc., 133 μm diameter gold pattern, 24 nm outer zone, 300 nm thickness), yielding a ≈30 nm full-width half-maximum lateral beam cross-section in the focal plane. To obtain such high spatial resolution, the centre part of the radially symmetric focused beam was blocked by a 40 μm diameter centre stop attached to the zone plate, resulting in a lateral beam cross-section in the form of an annulus of X-ray intensity [44] , [45] . The corresponding focused cone of X-rays had an incident angle spread of ≈0.30°. The BaTiO 3 crystals ({100} surface) were rotationally oriented to the crystallographic Bragg diffraction condition of tetragonal b domains ((220) reflection), in a horizontal diffraction geometry. Diffraction peaks were recorded using a 2D area CCD detector (Princeton PIXIS-XF: 1024F, 1024 × 1024 pixels, 13 μm 2 pixel size). Geometrical calibration parameters (sample-detector distance, detector centring and orientation) were determined from diffraction off a purely tetragonal domain using the focused beam. CCD images were recorded using 1.8 s of detector exposure and background-corrected using a 1.8 s dark count image. Imaging of the sample was performed by stepwise lateral scanning of the X-ray zone plate relative to the sample using a hybrid optomechanical nanopositioning system, recording the diffraction image at each step. Simultaneous detection of element-specific X-ray fluorescence allowed for positioning with respect to reference silver markers patterned on the sample surface. The focal plane was unambiguously established to within ≈20 μm (the axial depth of focus) using the X-ray fluorescence signal of one of the patterned silver markers. To prevent in situ domain structure rearrangement due to surface charging effects, a thin 5 nm layer of gold was deposited on the BaTiO 3 crystal surfaces and short-circuited to the sample mount. The addition of this thin conducting layer had no detectable effect on the observed domain structure, as confirmed by SHG imaging. Band-excitation piezoresponse force microscopy BE-PFM experiments were performed on a Cypher AFM (Asylum Research) using Cr/Pt coated conductive tips (Multi-75E-G, Budget Sensors) at the Center for Nanophase Materials Sciences (CNMS) at Oak Ridge National Laboratory. Typical imaging scan sizes were 30 × 30 μm, divided into a grid of 256 × 256 points. An AC driving voltage of 1.0 V was used. Details of the BE-PFM technique can be found elsewhere [54] . The resonance of the piezoelectric response measured at each grid point was fitted using a simple harmonic oscillator model and analysed using a custom-written algorithm. Figure 5 plots corresponding images of fitted response parameters (PFM resonance amplitude and phase). FEM simulations of PFM response The finite element method (FEM) was utilized to model the piezoresponse in the PFM experiments [65] , [66] , using the commercial ANSYS software. In the present simulations, the tip was modelled as a truncated cone (tip height 10 μm, full cone angle 30°) with a circular contact area (50 nm) with the sample surface [66] . The BaTiO 3 sample was modelled in an XYZ reference frame as a rectangular slab of 8 × 8 × 1 μm. A decoupled approximation was assumed [65] , [66] , [67] , [68] ; first, the electric field distribution in the sample was calculated, which was then used as input in the subsequent calculation of the piezoresponse. For different polarization rotation values, the latter used appropriate dielectric and piezoelectric property tensors extracted from the multi-domain phase-field simulations. The elastic properties of the monoclinic domain were assumed to be the same as that for tetragonal BaTiO 3 (ref. 69 ). A constant electric voltage of +1 V was applied to the tip surface, and the bottom surface of the sample slab was fixed to 0 V. In addition, the surface displacements ( U X , U Y and U Z ) were confined to 0 at the bottom of the sample (clamped bottom surface). The meshing was adjusted fine enough to yield results independent of the meshing size. Effective piezoelectric coefficients were estimated by linear multiplication of the FEM computed in-plane displacement in tetragonal b domains (using property tensors from multi-domain phase-field simulations) by the appropriate ratios of VPFM amplitudes (that is, U i ratios are taken the same as the corresponding VPFM amplitude ratios in the same scan). Calculation of material properties For the spatial property map calculations, the sets of local electric field ( E i ( x )) and stress ( σ ij ( x )) components at each spatial position x in the stabilized multi-domain structure (298 K, see Fig. 1c ) were extracted, with each set applied as external control parameters to a single BaTiO 3 domain in an independent single-domain simulation. Extracted local electric field components were multiplied by a factor of 0.5 to ensure an equivalent electrostatic energy contribution in the single domain simulations (where the electric field is treated as external, rather than internal). This approach allowed for the evaluation of the intrinsic properties of the domains stabilized in the multi-domain structure. Spatial maps of these local intrinsic properties were reconstructed using the grid site vectors x . Converse piezoelectric coefficients (in Voigt notation) were obtained from thermodynamic calculations using [70] : where ε 0 is the vacuum permittivity, and the piezoelectric coupling coefficient g ij is calculated from the Gibbs free energy G as: The dielectric susceptibility, defined as χ ij = η ij −1 , is calculated through the dielectric stiffness: Finally, all applied and calculated properties were transformed into the system of local symmetry coordinates (1,2,3), defined in analogy to the standard crystal physics axes adopted for tetragonal BaTiO 3 (ref. 42 ); at each grid site x the local 3 axis is assigned to the direction of the largest absolute XYZ component of the polarization P S (always in the XY-plane in our quasi-2D simulations), the local 1 axis is orthogonal to 3 and always along Z , and the local 2 axis is assigned to the in-plane direction orthogonal to 3, complementing the orthogonal right-handed coordinate system. How to cite this article: Lummen T. T. A. et al. Thermotropic Phase Boundaries in Classic Ferroelectrics. Nat. Commun. 5:3172 doi: 10.1038/ncomms4172 (2014).